Room-temperature air-stable spin transport in bathocuproine-based spin valves Organic semiconductors, characterized by weak spin-scattering mechanisms, are attractive materials for those spintronic applications in which the spin information needs to be retained for long times. Prototypical spin-valve devices employing organic interlayers sandwiched between ferromagnetic materials possess a figure of merit (magnetoresistance (MR)) comparable to their fully inorganic counterparts. However, these results are a matter of debate as the conductivity of the devices does not show the expected temperature dependence. Here we show spin valves with an interlayer of bathocuproine in which the transport takes place unambiguously through the organic layer and where the electron spin coherence is maintained over large distances (>60 nm) at room temperature. Additionally, the devices show excellent air stability, with MR values almost unaltered after 70 days of storage under ambient conditions, making bathocuproine an interesting material for future spintronic applications. In spintronics applications, the information is carried not only by the electron charge, but also by the electron spin [1] . One of the simplest spintronic devices is the spin valve (SV), composed of two ferromagnetic metals (FMs) separated by a non-magnetic interlayer. In such a device, one of the FM is used to inject electrically a spin-polarized current into the non-magnetic interlayer, and the other one to detect it. The detection occurs via a change in the electrical resistance of the device depending on the relative alignment of the magnetization of the two FMs, achievable in a magnetic field sweep [2] , [3] . This effect is characterized by the magnetoresistance (MR) ratio, defined as MR=( R p − R ap )/ R ap , and takes place only if the spin information is not lost across the interlayer material [4] . Therefore, materials with long spin lifetime are extremely attractive for spintronics, because they offer the possibility to retain the spin information over long distances and perform advanced spin manipulations. In this context, organic semiconductors have emerged as promising materials for spintronics [5] . Their spin-scattering mechanisms are extremely weak, and ultrahigh spin lifetimes (in the μs range) have been measured [6] . Organic spintronics is now an active research field, and different molecules have been used as interlayers in SV-like structures [7] , [8] , [9] , [10] , [11] , [12] , [13] , [14] , [15] . The measurement of MR in these devices is taken as the demonstration of the spin transport across the organic layer, which in some cases is very thick [7] , [9] (>100 nm). In addition to the long spin lifetimes, it has been noticed that the combination of molecules and FM offers other intriguing possibilities for spintronics. For instance, devices with novel functionalities have been demonstrated by exploiting properties of the semiconducting molecules, such as light emission [16] , electrical bistability [17] and hot electron filtering [18] . Furthermore, reaction at a molecule/FM interface can result in interfacial states [19] , [20] with modified energetics and spin polarization. These new states are crucial for the operation of devices, as they can cause inversion or enhancement of MR [12] , as well as form FM organometallic compounds that behave as spin filters [15] . There are two main issues that remain a matter of controversy in organic spintronics. First, the temperature dependence of the resistance of most organic SVs is weak [7] , [8] , [9] , [10] , [11] , [12] , [13] , [14] , [15] , [16] , [17] , resembling more the behaviour of a tunnel junction than the temperature-activated transport typical of organic films [21] . Therefore, the question rises whether the SVs are actually probing the properties of the organics, or they are prone to artifacts coming from the interpenetration of the top metal contact into the organic layer. Second, a thin AlO x seed interlayer is often inserted between the organics and the FM contact [8] , [10] , [11] , [13] , [14] , [22] . Such a layer has been shown to enhance the spin polarization of the current injected into the organic [8] , but its effect on the transport properties remains unclear. In this article, we present results on SVs based on bathocuproine (BCP) spacer layers of various thickness (from 5 to 60 nm), which show both high MR at room temperature and excellent stability under air atmosphere. We employ different AlO x seed layers – either leaky or non-leaky – and we show that a different transport mechanism is relevant in each case. In particular, when the AlO x seed layer is non-leaky and forms a true inorganic tunnel barrier, the device resistance is extremely high even at room temperature and has weak (tunnelling-like) temperature dependence. In this case, MR is only measured in SVs with thin BCP layers, as expected for transport in the tunnelling regime. Instead, when leaky seed layers are employed, a strong temperature dependence of the junction resistance is found, demonstrating that the charge transport takes place in the organic layer. Under these conditions, MR is measured even for thick BCP layers (up to 60 nm). These devices also show excellent air stability, with MR almost unaltered after 70 days of storage under ambient conditions. Materials and sample fabrication BCP is an organic semiconductor (inset in Fig. 1a ) commonly used in many organic devices, such as organic solar cells and organic light-emitting diodes [23] , [24] . BCP has similarities to the Tris-(8-hydroxyquinoline) aluminium (Alq 3 ), which is one of the most commonly employed materials in organic-based spintronic devices. Both materials have similar lowest unoccupied molecular orbital (LUMO, ~3.2 eV, Fig. 1b ) and behave as electron transport and hole-blocking materials because of their large band gap. Furthermore, BCP is air stable, allowing the operation of devices at room temperature in ambient conditions. Finally, BCP is commercially available with high purity (99.99%), a crucial aspect for the reliable systematic fabrication and investigation of organic devices. 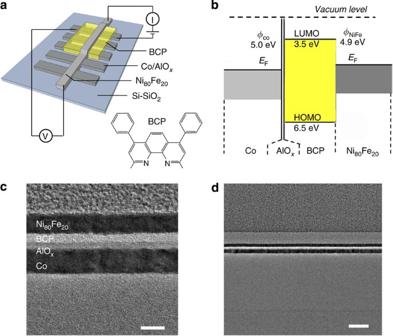Figure 1: Multilayer sample schematics and microscopic characterization. (a) Schematic representation of the sample fabricated in this paper and molecular structure of BCP. (b) Rigid energy diagram for the Co/AlOx/BCP/Ni80Fe20stack. (c) and (d) TEM cross-sectional images of a BCP-based SV structure. The layers of the junction, from bottom to top, are Co, AlOx, BCP and Ni80Fe20, respectively. Note that this specific sample has been produced with a thicker AlOxlayer than the one commonly used for transport measurements with the aim of easily identifying the different materials in the TEM. Scale bars incanddrepresent 10 and 50 nm, respectively. Figure 1: Multilayer sample schematics and microscopic characterization. ( a ) Schematic representation of the sample fabricated in this paper and molecular structure of BCP. ( b ) Rigid energy diagram for the Co/AlO x /BCP/Ni 80 Fe 20 stack. ( c ) and ( d ) TEM cross-sectional images of a BCP-based SV structure. The layers of the junction, from bottom to top, are Co, AlO x , BCP and Ni 80 Fe 20 , respectively. Note that this specific sample has been produced with a thicker AlO x layer than the one commonly used for transport measurements with the aim of easily identifying the different materials in the TEM. Scale bars in c and d represent 10 and 50 nm, respectively. Full size image The cross-bar geometry of the vertical SV, with a structure of Co (11 nm)/AlO x /BCP(5–60 nm) /Ni 80 Fe 20 (11 nm) (from bottom to top, see Fig. 1a ) was deposited through shadow masks in a ultrahigh vacuum dual chamber evaporator. Different durations of the plasma treatment have been employed in different samples in order to obtain either a leaky or a non-leaky AlO x barrier. In every chip, two junctions are left with only the AlO x layer and without organic material between the two FMs, these junctions being used as a reference for the characterization of the AlO x layer. As displayed in Fig. 1c , the cross-sectional transmission electron microscopy (TEM) images of a 5 nm-thick BCP SV show the presence of sharp interfaces and long-range homogeneity in all the device layers ( Fig. 1c,d ). See Methods for details on the TEM sample preparation and imaging. The low-temperature and rate-controlled fabrication strategy employed (see Methods) prevents the diffusion of the top metal electrode into the BCP layer, as evidenced by the clear and sharp contrast at the BCP/NiFe interface (see Fig. 1c and Supplementary Fig. S1 ) [25] . Inorganic reference devices We distinguish between leaky and non-leaky AlO x barrier primarily on the basis of the temperature dependence of the resistance of the reference junctions. All along this manuscript, we calculate the junction resistances using the d I /d V around zero bias. As shown in Fig. 2a , the resistance of the purely inorganic non-leaky AlO x junction slightly increases when lowering the temperature, as expected for a continuous tunnel barrier [26] . On the contrary, the junction with leaky AlO x has by far lower resistance than the non-leaky junction, and the temperature-dependence measurements show metal-like behaviour (see Fig. 2a ). Moreover, the SVs with non-leaky AlO x barrier have MR around 2% at room temperature, whereas the samples with leaky AlO x display no MR (not shown). 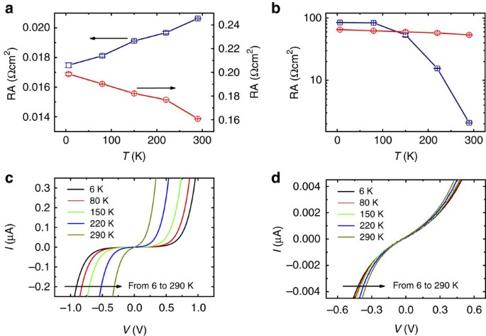Figure 2: Temperature-dependent resistance and current–voltage measurements. Comparison of the temperature dependent resistance of (a) Co/AlOx/Ni80Fe20junction and (b) Co/AlOx/BCP/Ni80Fe20junction based on leaky (blue squares) or non-leaky (red circles) AlOxbarriers. The error bars correspond to the distribution of the measured data from three junctions on same chip. Temperature dependence ofI–Vcurves from 5 nm BCP-based SVs with (c) leaky AlOxlayer and (d) non-leaky AlOxlayer. These measurements are carried out in vacuum. Figure 2: Temperature-dependent resistance and current–voltage measurements. Comparison of the temperature dependent resistance of ( a ) Co/AlO x /Ni 80 Fe 20 junction and ( b ) Co/AlO x /BCP/Ni 80 Fe 20 junction based on leaky (blue squares) or non-leaky (red circles) AlO x barriers. The error bars correspond to the distribution of the measured data from three junctions on same chip. Temperature dependence of I – V curves from 5 nm BCP-based SVs with ( c ) leaky AlO x layer and ( d ) non-leaky AlO x layer. These measurements are carried out in vacuum. Full size image Charge carrier transport of BCP devices We focus now on the properties of the BCP-based devices. Figure 2b shows the temperature-dependence of the resistance of two Co/AlO x /BCP(5 nm)/Ni 80 Fe 20 junctions, which are identical apart from the fact that one is based on a leaky AlO x barrier and the other one on a non-leaky one. The corresponding I – V traces are displayed in Fig. 2c,d , respectively. Despite the very similar fabrication recipe, the transport properties of the two samples are very different. First, the room temperature resistance of the SV with the non-leaky barrier is extremely high (>100 MΩ). Second, the temperature dependence of the resistance for the two different devices is substantially different, suggesting that distinct charge transport mechanisms are involved in either case and shedding light on the role of the AlO x layer in organic SVs. The temperature dependence of the non-leaky-AlO x BCP junctions is weak, with a 15% resistance change between room temperature and 6 K. Such temperature dependence has been reported for similar devices based on other molecular species grown on non-leaky AlO x layers [8] , [10] , [11] , [14] , [22] , and is typically taken as demonstration of direct and multistep tunnelling [14] . We believe that the presence of the non-leaky AlO x layer does not allow the injection of the current from the bottom metal electrode into the LUMO of the BCP layer. The non-leaky AlO x and the 5 nm BCP film behave jointly as an insulating barrier, so that only a tunnelling current can flow between the electrodes, either via a direct or a multistep tunnelling mechanism. In the device shown in Fig. 1f , the nominal barrier thickness is 6.5 nm, very thick compared with the typical tunnelling regime. For this reason, the device resistance is above 100 MΩ even at room temperature. In junctions with 10 nm thick BCP layers, the resistance was extremely high (in the TΩ range), with almost no detectable current below 1 V. On the contrary, the resistance of the sample with the leaky seed layer displays strong temperature dependence in the range between 300 and 100 K, reaching a plateau below 100 K. This behaviour is commonly observed in devices based on amorphous organic semiconductors with interface-limited charge injection [21] . We are therefore confident that the leaky AlO x layer allows the charge injection into the organic layer so that the transport takes place in the LUMO of the semiconductor. To the best of our knowledge, such temperature dependence has not been observed in organic SVs showing MR. In most reported organic spintronics experiments, an optimized AlO x tunnel barrier seed layer was employed between the ferromagnetic bottom electrode and the organic semiconductor, explaining why an extremely high resistance with weak temperature dependence was typically measured [8] , [10] , [11] , [14] , [22] . It is worth to mention that an AlO x layer is known to generate metallic filaments through almost all organic layers [27] . Such an AlO x layer would be extremely similar to the leaky AlO x barrier we employ. The metallic filaments are driven by an applied bias voltage and can cause dramatic resistance changes [28] , [29] . In our devices, the I – V characteristics are extremely stable in the voltage range between −0.5 and 0.5 V or −1 and 1 V, remaining unaltered even after 500-times or 1,000-times voltage loops, respectively (see Fig. 3a,b ). Furthermore, the current flowing continuously at a fixed bias does not show any sudden change for measurement times over 24 h (see Supplementary Fig. S2 ). We therefore argue that the presence of filaments does not affect the transport through our devices in the voltage range we are interested in. Concomitantly, the spin transport experiments are performed with an applied voltage well below 1 V, typically around 10 mV. 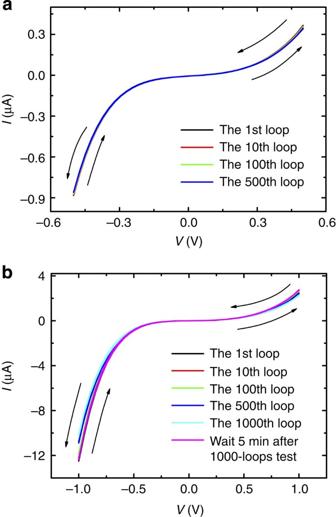Figure 3:Current–voltage loop measurements of 5 nm thick BCP SV with leaky AlOxbarrier. A current–voltage loop represents the current measured while the voltage is swept from negative to positive and back again to negative. (a) 500 current–voltage loops measurements with a voltage range from −0.5 to 0.5 V (b) 1,000 current–voltage loops measurement with a voltage range from −1 to 1 V. These measurements are carried out in vacuum. Figure 3: Current–voltage loop measurements of 5 nm thick BCP SV with leaky AlO x barrier. A current–voltage loop represents the current measured while the voltage is swept from negative to positive and back again to negative. ( a ) 500 current–voltage loops measurements with a voltage range from −0.5 to 0.5 V ( b ) 1,000 current–voltage loops measurement with a voltage range from −1 to 1 V. These measurements are carried out in vacuum. Full size image Room-temperature spin transport of BCP devices We focus now on the magnetic properties of our BCP-based SVs, starting from the ones with a non-leaky AlO x . As we discussed above, for this set of samples we expect tunnelling to be the main transport mechanism and a MR signal should be measurable in devices with very thin BCP layers. The reference junction shows a 2% MR ( Fig. 4a ; Supplementary Fig. S3 ), which is far lower than the recorded for the non-leaky-AlO x SV with 5 nm BCP (which displays 7% MR) in the same chip (see Fig. 4b ). The devices become extremely resistive when the BCP thickness is increased above 10 nm, preventing the measurement of any clear MR signal. Long-distance spin transport cannot be achieved in the devices with non-leaky AlO x layer, because the tunnelling mechanism itself is not compatible with long-distance charge transport. 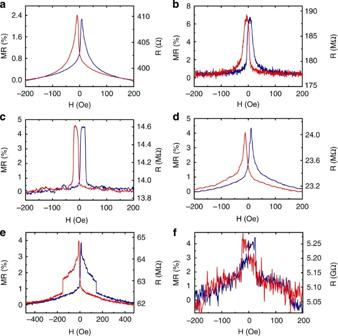Figure 4:Room-temperature MR curves of the BCP-based SVs under vacuum. (a) Reference SV (without BCP) with non-leaky AlOx, (b) 5-nm-BCP SV with non-leaky AlOx, (c) 5-nm-BCP SV with leaky AlOx, (d) 10-nm-BCP SV with leaky AlOx, (e) 30-nm-BCP SV with leaky AlOxand (f) 60-nm-BCP SV with leaky AlOx. The blue lines and red lines represent the MR value while the voltage is swept from negative to positive and back from positive to negative, respectively. All these measurements are carried out in vacuum. Figure 4: Room-temperature MR curves of the BCP-based SVs under vacuum . ( a ) Reference SV (without BCP) with non-leaky AlO x , ( b ) 5-nm-BCP SV with non-leaky AlO x , ( c ) 5-nm-BCP SV with leaky AlO x , ( d ) 10-nm-BCP SV with leaky AlO x , ( e ) 30-nm-BCP SV with leaky AlO x and ( f ) 60-nm-BCP SV with leaky AlO x . The blue lines and red lines represent the MR value while the voltage is swept from negative to positive and back from positive to negative, respectively. All these measurements are carried out in vacuum. Full size image The situation is different for the leaky-AlO x BCP junction, where we believe that the transport takes place in the molecular levels of BCP. We measure MR for different thicknesses of the BCP layer, as shown in Fig. 4c–f for 5, 10, 30 and 60 nm of BCP, respectively. Even for the case of the 60-nm-thick BCP film the MR signal is still clearly distinguishable, although the curve becomes noisy because of the high junction resistance (in the GΩ range). The differences in the transport mechanisms present in the devices with either leaky or non-leaky AlO x barrier are analysed in detail in the following section. 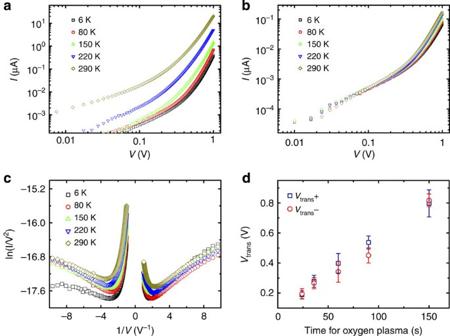Figure 5: Analysis of the current–voltage properties of BCP SVs. aandbare the log–log plots of current–voltage curves of BCP SVs with leaky and non-leaky AlOx, respectively. (c) ln(I/V2) versus 1/Vplots of the 5-nm-BCP junction with non-leaky AlOx. (d) Time for oxygen plasma versusVtransof the BCP-based junctions with non-leaky AlOxlayers.Vtrans+corresponds to electrons injected from the Co;Vtrans– to electrons injected from Ni80Fe20. The error bars correspond to the distribution of the measured data of five devices on the same chip. Figure 5a shows the log–log plot of the I – V traces of BCP SVs with leaky AlO x . Every I – V trace shows two different voltage ranges, in which the current increases following a power-law dependence (linear in the log–log plot) but with different exponents ( Fig. 5a ). These two different regimes following a power law at low and high bias correspond to an ohmic conduction and a field emission regime, respectively [30] , [31] . The room-temperature current scales linearly with voltage in the low bias regime which is consistent as well with an ohmic hopping conduction (see Fig. 5a ) [30] , [31] . In our experimental data, we can observe three distinct features of the temperature-dependent I – V traces of the devices with leaky AlO x barrier that are typical of amorphous organic layers with hopping transport [21] . First, the current – at constant bias – increases as the temperature is increased (also see Fig. 2b ). Second, the voltage at which the power-law exponents change is temperature dependent (see Supplementary Fig. S4a ). Third, in the log–log plot, the slope of the power law at high applied voltages decreases when temperature increases (see Supplementary Fig. S4b ). On the other hand, none of the characteristics outlined above and related with the charge transport in amorphous organic layer, is found in the devices with non-leaky AlO x ( Fig. 5b ). In this case, the results are better described by a tunnelling framework characterized by weak temperature dependence. Figure 5: Analysis of the current–voltage properties of BCP SVs. a and b are the log–log plots of current–voltage curves of BCP SVs with leaky and non-leaky AlO x , respectively. ( c ) ln( I / V 2 ) versus 1/ V plots of the 5-nm-BCP junction with non-leaky AlO x . ( d ) Time for oxygen plasma versus V trans of the BCP-based junctions with non-leaky AlO x layers. V trans +corresponds to electrons injected from the Co; V trans – to electrons injected from Ni 80 Fe 20 . The error bars correspond to the distribution of the measured data of five devices on the same chip. Full size image In order to gain more insight on the role of the AlO x tunnel barrier in the transport through the BCP molecular layer, we analyse the I – V traces of the devices with non-leaky AlO x via the so-called voltage transition spectroscopy [32] . According to this method, the barrier energy profile of a tunnel junction changes from trapezoidal to triangular as the bias increases, leading to different dependences in the I – V characteristics. The voltage at which the barrier changes its shape appears as an inflection point V trans in a plot of ln( I/V 2 ) versus 1/ V (see Fig. 5c ) [30] , [31] , [32] . As shown in Fig. 5c , the V trans of the BCP SV with non-leaky AlO x shows a weak temperature dependence, which means the barrier height of AlO x /BCP double layer is not much sensitive to the temperature. However, by changing the plasma exposure time of the Al during the device fabrication, the absolute value of V trans , that is, the barrier height, increases with the duration of oxygen plasma (see Fig. 5d ). Our interpretation of this dependence is that a continuous tunnel barrier is formed when a relatively long plasma oxidation time is employed. By decreasing the oxygen plasma time, the barrier height becomes lower, eventually reaching the point where the transport deviates from the standard tunnelling framework (at t =24 s, V =0.2 V). This point corresponds to our definition of the transition from a non-leaky to a leaky barrier. In the leaky barrier regime, the barrier height is no longer dominated by the AlO x , but rather by the energy mismatch between the Fermi level of metallic electrodes and the LUMO of BCP. Then, the transport mechanism follows the typical behaviour of an amorphous organic semiconductor, as highlighted above. Turning back again to the spin transport properties of the BCP-based SVs, besides the large room-temperature MR signals they also present excellent air-atmosphere stability. 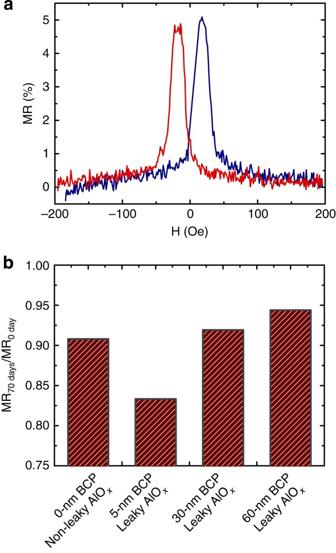Figure 6: Air-stable MR of BCP SVs. (a) 5-nm-BCP SV with leaky AlOxbarrier tested under air atmosphere at room temperature. The blue line and red line represent the MR value while the voltage is swept from negative to positive and back again to negative, respectively. (b) room-temperature MR changes of SVs with 0 (with non-leaky AlOx), 5, 30 and 60 nm (all with leaky AlOx) after stored in air for 70 days. Figure 6a shows the MR measured in air for the same samples of Fig. 4c . By comparing the different graphs, it is clear that the BCP-based SVs display similar properties when measured in vacuum and in air, both in terms of MR values and of signal shape. Even after a 70-day storage in air atmosphere, BCP-based junctions display only slight changes on MR values (see Fig. 6b ). This figure shows that the MR of SVs with BCP thickness of 5, 30 and 60 nm decreased by 17, 8 and 5.5%, respectively, and the reference junction with 1.5 nm non-leaky AlO x show a 9% decrease after the 70-days storage in air atmosphere. The stability of the SVs with thicker BCP layers stored in air is hence also better than the inorganic SVs (1.5 nm non-leaky AlO x ). As the Ni 80 Fe 20 top electrodes in different samples show similar air-stability and the junction resistances do not change significantly after 70-days of storage in air, we hypothesize that the decrease of MR is most probably related to the oxidation of the Co bottom electrode. Following storage in air for 70 days, the resistance of the Co line in SVs with 5 nm BCP increases >10%, whereas for SVs with thicker BCP layer (30 and 60 nm), the Co line shows almost no change on resistance. We can explore as well the changes in the anisotropic MR of Co, which should have a relation with the changes in the MR of the devices. In order to study the effectiveness of the BCP layer protection, we fabricated a series of samples with a Co/AlO x /BCP structure, with different BCP thicknesses and no Ni 80 Fe 20 top electrodes. After storage in air for 1 month, the anisotropic MR of the Co lines decrease to 70% (0 nm BCP), 63% (5 nm), 80% (30 nm) and 83% (60 nm) (see Supplementary Figs S5 and S6 ), which follow the same trend as the MR in the full junction (in Fig. 6b ). This fact confirms that the samples covered with thicker BCP layer present an improved air stability. Figure 6: Air-stable MR of BCP SVs. ( a ) 5-nm-BCP SV with leaky AlO x barrier tested under air atmosphere at room temperature. The blue line and red line represent the MR value while the voltage is swept from negative to positive and back again to negative, respectively. ( b ) room-temperature MR changes of SVs with 0 (with non-leaky AlO x ), 5, 30 and 60 nm (all with leaky AlO x ) after stored in air for 70 days. Full size image In conclusion, we have produced and characterized SVs based on the organic semiconductor BCP. In two sets of devices, different AlO x seed layers have been employed, that we distinguish between ‘leaky’ and ‘non-leaky’ on the basis of the temperature dependence of their resistance. For the devices with non-leaky seed layer, the main charge transport mechanism is tunnelling, and consequently MR is measured only for extremely thin BCP films (5 nm). By contrast, for devices with leaky AlO x layer, the transport takes place into the BCP film, and MR is measured up to a thickness of 60 nm. Our results shed some light on the role of the AlO x layer on the transport mechanism of the whole junction. Furthermore, they might explain why the measurement of MR was always accompanied by a weak temperature dependence of the device resistance in devices with an optimized AlO x layer [8] , [10] , [11] , [13] , [14] , [22] , not matching with the expected behaviour of the organic layer. Finally the BCP-based SVs have shown excellent air-condition stability in terms of device performance even after long time (more than 70 days), in this respect outperforming most of the reported organic SVs. The observation of air-stable room-temperature spin transport in our BCP-based SVs is of great importance for both scientific research and future industrial interest in organic spintronics. Sample fabrication Co/AlO x /BCP/Ni 80 Fe 20 vertical SVs have been fabricated in situ in a ultrahigh vacuum dual chamber evaporator (base pressure <10 −9 mbar). The junction areas range from 200 × 200 μm 2 to 500 × 200 μm 2 . In all samples, five 11-nm-thick Co lines are deposited as bottom electrodes. Then, a 1.5-nm-thick Al layer was deposited on top and was oxidized in situ by oxygen plasma. By controlling the time of the oxidized process, we could obtain leaky and non-leaky AlO x . The BCP layers have been deposited onto the AlO x though a shadow mask designed to cover only three of the five bottom contacts. Therefore, two Co lines are left only covered by AlO x and employed as reference junction in our study. Finally, an 11-nm-thick Ni 80 Fe 20 line has been deposited in cross direction as the top electrode. The metals (Co, Al and Ni 80 Fe 20 ) are purchased from Lesker (of 99.95% purity), and have been deposited by e-beam in one of the chambers with a deposition rate of ~1 Å s −1 (the first 2 nm of Ni 80 Fe 20 has been deposited with a lower rate of ~0.1 Å s −1 for protecting the organic layer). Liquid nitrogen has been used to cool down the sample during the deposition of metals for obtaining smooth metal films. The BCP has been purchased from Aldrich with a purity of 99.99% (sublimed grade, used without further purification), and has been evaporated in another chamber from a Knudsen cell at a rate of 1.8 Å s −1 . Experimental set-up TEM study was performed on Titan G2 60-300 (FEI, Netherlands) TEM operated at 300 kV. Cross-sectional samples for TEM were prepared by standard Focused Ion Beam method using Helios Nanolab (FEI, Netherlands) DualBeam instrument. In order to protect the surface layer and the subsurface organic layer during cutting, 50 nm of Pt was deposited on the surface by electron-beam-induced deposition at 2 kV acceleration voltage and 100 pA beam current, followed by 150 nm of Pt at 5 kV and 2.7 nA, followed by 2 um of Pt deposited by ion-beam-induced deposition. Electrical characterization was performed under vacuum (or in air atmosphere) with a magnetic-field-equipped Lakeshore probe station in which the temperature could vary from 6 to 300 K. A Keithley 4,200 semiconductor analyser system has been used to record I – V and MR curves. For the time-dependent air-stability tests, the BCP SVs were stored in dark and in air. Junctions grown in the same chip have extremely similar transport characteristics, whereas there are small chip-to-chip variations due to unavoidable variables in the fabrication. Atomic force microscope images were recorded in tapping mode with an Agilent AFM. The root-mean-squared roughness (calculate from 5 × 5 μm 2 AFM images) of 5, 30 and 60 nm BCP layers covering the Co/AlO x electrodes is 0.22, 0.74 and 1.12 nm, respectively. Model The model employed herein to analyse the temperature-dependence of the tunnelling barrier transmission in the discussion section was deduced from Simmons approximation, and could be described as follows [32] : where d is the barrier width, m e is the electron effective mass, ϕ is the barrier height and ħ is the Planck constant. In this model, the change of transport mechanism from direct tunnelling to field emission could be reflected in a plot of ln( I / V 2 ) versus 1/ V . With this plot, we can get the value of V trans at which the tunnelling barrier changes from trapezoidal to triangular. How to cite this article: Sun, X. et al. Room-temperature air-stable spin transport in bathocuproine-based spin valves. Nat. Commun. 4:2794 doi: 10.1038/ncomms3794 (2013).